Early-onset metabolic syndrome in mice lacking the intestinal uric acid transporterSLC2A9 Excess circulating uric acid, a product of hepatic glycolysis and purine metabolism, often accompanies metabolic syndrome. However, whether hyperuricaemia contributes to the development of metabolic syndrome or is merely a by-product of other processes that cause this disorder has not been resolved. In addition, how uric acid is cleared from the circulation is incompletely understood. Here we present a genetic model of spontaneous, early-onset metabolic syndrome in mice lacking the enterocyte urate transporter Glut9 (encoded by the SLC2A9 gene). Glut9-deficient mice develop impaired enterocyte uric acid transport kinetics, hyperuricaemia, hyperuricosuria, spontaneous hypertension, dyslipidaemia and elevated body fat. Allopurinol, a xanthine oxidase inhibitor, can reverse the hypertension and hypercholesterolaemia. These data provide evidence that hyperuricaemia per se could have deleterious metabolic sequelae. Moreover, these findings suggest that enterocytes may regulate whole-body metabolism, and that enterocyte urate metabolism could potentially be targeted to modulate or prevent metabolic syndrome. Metabolic syndrome is a complex multifactorial disease that afflicts two in five adults in the U.S. alone [1] , and scores more worldwide. Observations over the prior two decades demonstrated increased metabolic syndrome, type 2 diabetes mellitus and cardiovascular morbidity in hyperuricaemic subjects [2] , [3] , and that serum uric acid levels independently predict diabetes, fatty liver and metabolic syndrome [2] . Work in rodent models further mechanistically implicated uric acid in fructose-induced metabolic syndrome [4] , although some controversy over the exact physiological function of urate (the predominant form of uric acid at physiological pH) remains [5] , [6] . Elucidating how urate is removed from the circulation may nevertheless have broad individual and public health implications. Approximately 60–70% of circulating uric acid clearance occurs in the kidney and the other 30–40% is cleared via intestinal enterocytes [7] , although the enterocyte may become the primary excretory pathway in renally insufficient patients [8] (for example, in patients with diabetes, hypertension or cardiorenal disease). Recent data suggest that defective extrarenal clearance is a common cause of hyperuricemia [9] , yet few studies address enterocyte urate-handling mechanisms [9] , [10] , [11] , and none address endogenous urate clearance mechanisms as effectors of mammalian metabolism. The putative enterocyte urate transporters—BCRP/ABCG2 (and potentially SLC17A4/NPT5) are apical transporters [10] , [11] , whereas a basolateral transporter has not been identified. Therefore, it was unresolved how uric acid flux occurred down its gradient from the blood into the enterocyte cytoplasm before excretion in the stool. Recent data in humans and in rodents identified GLUT9/Glut9 as a high-capacity urate transporter [12] , [13] , the deletion of which alters urate homeostasis in a tissue-specific manner [14] , [15] . Furthermore, Glut9 is a basolateral and apical membrane transporter in other polarized epithelial cell types [12] . Thus, we examined GLUT9 localization, cellular function and role in urate homeostasis in the murine intestine. Here we show that Glut9 is localized to the apical and basolateral enterocyte membranes, and that enterocyte-specific Glut9 deficiency impairs enterocyte urate transport. Concomitant with these urate clearance defects, enterocyte Glut9-deficient mice develop hyperuricaemia, hyperuricosuria and early-onset metabolic syndrome—hypertension, dyslipidaemia, hyperinsulinaemia and hepatic fat deposition—which is partly mitigated by ad lib administration of the xanthine oxidase inhibitor, allopurinol. These results suggest that Glut9 regulates enterocyte urate clearance, and that enterocyte Glut9 deficiency may have deleterious metabolic sequelae. Expression and localization of enterocyte Glut9 Immunoblot analysis demonstrated that Glut9 was abundantly expressed in intestine ( Fig. 1a ), highly in the jejunum and ileum ( Fig. 1b ), the segments of the intestine that perform the majority of urate excretion [8] , [10] . Confocal immunofluorescence microscopy of fixed mouse intestine revealed Glut9 localized predominantly to the basolateral enterocyte membrane with some apical staining ( Fig. 1c ). 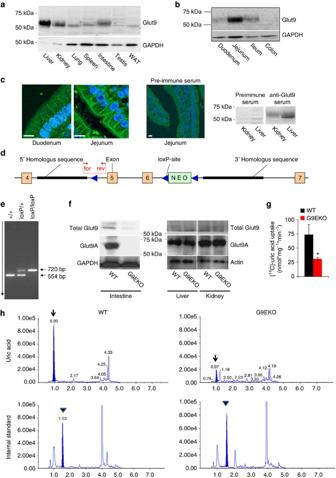Figure 1: Characterization of intestinal Glut9 and genetic deletion of enterocyte SLC2A9. (a) Immunoblotting against full-length Glut9 in murine tissue. (b) Small-bowel segment-specific Glut9 immunoblotting. (c) Left, confocal immunofluorescence microscopy demonstrating basolateral and apical Glut9 localization in duodenum and jejunum. Middle, jejunal immunostaining with pre-immune serum. Scale bar, 10 μm. Right, specificity of total Glut9 antiserum versus pre-immune serum by liver and kidney lysate immunoblotting (d) Glut9-targeting construct used to generate mice harbouring floxedSLC2A9flanking exons 5 and 6. Forward and reverse (for/rev) genotyping primers flank the flox site adjacent to exon 5. (e) PCR bands depicting larger floxed (720 bp) and wild-type (WT) (554 bp) sequences. (f) Immunoblot of Glut9A in WT and G9EKO mouse whole intestine, liver and kidney lysate. (g) [14C]-uric acid uptake in purified villous enterocyte fractions from WT and G9EKO mice.n=5 per group.In vitroexperiment replicated thrice. *P<0.05 versus WT (two-tailedt-testing). Error bars represent s.e.m. (h) LC/MS analysis of stool from WT and G9EKO mice. Upper spectra—uric acid (arrows) elution. Lower spectra (arrowheads)—1-methyluric acid internal standard. Experiment replicated thrice. Figure 1: Characterization of intestinal Glut9 and genetic deletion of enterocyte SLC2A9. ( a ) Immunoblotting against full-length Glut9 in murine tissue. ( b ) Small-bowel segment-specific Glut9 immunoblotting. ( c ) Left, confocal immunofluorescence microscopy demonstrating basolateral and apical Glut9 localization in duodenum and jejunum. Middle, jejunal immunostaining with pre-immune serum. Scale bar, 10 μm. Right, specificity of total Glut9 antiserum versus pre-immune serum by liver and kidney lysate immunoblotting ( d ) Glut9-targeting construct used to generate mice harbouring floxed SLC2A9 flanking exons 5 and 6. Forward and reverse (for/rev) genotyping primers flank the flox site adjacent to exon 5. ( e ) PCR bands depicting larger floxed (720 bp) and wild-type (WT) (554 bp) sequences. ( f ) Immunoblot of Glut9A in WT and G9EKO mouse whole intestine, liver and kidney lysate. ( g ) [ 14 C]-uric acid uptake in purified villous enterocyte fractions from WT and G9EKO mice. n =5 per group. In vitro experiment replicated thrice. * P <0.05 versus WT (two-tailed t -testing). Error bars represent s.e.m. ( h ) LC/MS analysis of stool from WT and G9EKO mice. Upper spectra—uric acid (arrows) elution. Lower spectra (arrowheads)—1-methyluric acid internal standard. Experiment replicated thrice. Full size image Generation of mice lacking enterocyte Glut9 Given that Glut9 is the only reported basolateral urate transporter, we hypothesized that mice lacking Glut9 in enterocytes would have impaired enteric urate handling. We thus generated enterocyte-specific Glut9-deficient mice by crossing mice harbouring a floxed SLC2A9 allele with mice overexpressing cre recombinase driven by the enterocyte-specific villin promoter ( Fig. 1d,e ). vil -Cre/ SLC2A9 fl/fl (G9EKO) mice were live-born in Mendelian ratios, were fertile and had no gross morphologic defects ( Table 1 ). Immunoblotting confirmed deficiency of total Glut9A and total Glut9 protein in G9EKO small-bowel lysates ( Fig. 1f and Supplementary Figs 1 and 2 ). Isolated villous enterocytes from G9EKO mice exhibited an ~65% [ 14 C]-urate uptake defect versus wild-type (WT) enterocytes when compared with mice expressing vil- Cre with WT SLC2A9 alleles (hereafter referenced as ‘WT’ mice) ( Fig. 1g ). Congruent with these findings, liquid chromatography–mass spectrometry (LC/MS) of stool extracts revealed significantly decreased stool urate concentrations in G9EKO mice versus WT mice ( Fig. 1h ). Together, these results suggested impaired enterocyte uptake and efflux into stool in G9EKO animals. Table 1 Basic morphometric parameters in wild-type (WT) and G9EKO mice. Full size table Physiological consequences of impaired enterocyte urate clearance We next examined physiological consequences of impaired enterocyte urate efflux in mice fed standard rodent chow (Picolab #5053: 25% protein, 13% fat and 62% carbohydrate). Uricase-based urate determinations further revealed significantly higher uric acid concentrations in both serum and urine in G9EKO mice ( Fig. 2a,b ). Body composition analysis by EchoMRI revealed significantly elevated body fat mass and fat percentage ( Fig. 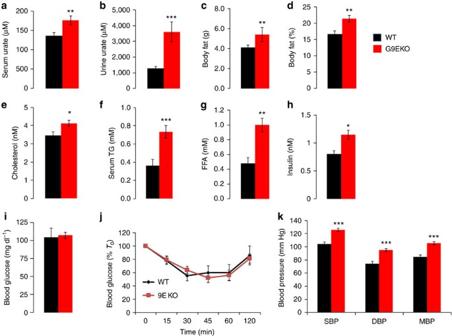Figure 2: Physiological consequences of enterocyte Glut9 deficiency. (a,b) Serum (n=9, 16) and urine (n=13, 12) uric acid concentration in fasting 6–8-week-old mice. (c,d) EchoMRI analysis of fat mass and percentage fat (n=19, 10). (e–i) Plasma cholesterol (n=6, 5), triglycerides, free fatty acids, insulin (n=5, 4) and glucose in fasting WT and G9EKO mice. (j) Insulin tolerance testing in 4-h fasting mice (n=6, 22). (k) Systolic (SBP), diastolic (DBP) and mean (MBP) blood pressure in non-fasting WT mice and G9EKO (n=9, 17). *P<0.05, **P<0.01 and ***P<0.001 versus WT (two-tailedt-testing). Error bars represent s.e.m. 2c,d ) despite higher resting energy expenditure as determined by indirect calorimetry in G9EKO mice ( Table 2 ). Plasma analysis revealed G9EKO mice had significantly elevated total cholesterol, free fatty acids and triglycerides ( Fig. 2e–g ). Some evidence of early insulin resistance was observed, with an approximately 40% elevation in fasting plasma insulin in G9EKO mice ( Fig. 2h ) in context of normal fasting blood glucose ( Fig. 2i ) and insulin tolerance testing ( Fig. 2j ). Tail-cuff plethysmography in unanaesthetized G9EKO mice demonstrated significant baseline hypertension when compared with WT mice ( Fig. 2k ). Figure 2: Physiological consequences of enterocyte Glut9 deficiency. ( a , b ) Serum ( n =9, 16) and urine ( n =13, 12) uric acid concentration in fasting 6–8-week-old mice. ( c , d ) EchoMRI analysis of fat mass and percentage fat ( n =19, 10). ( e – i ) Plasma cholesterol ( n =6, 5), triglycerides, free fatty acids, insulin ( n =5, 4) and glucose in fasting WT and G9EKO mice. ( j ) Insulin tolerance testing in 4-h fasting mice ( n =6, 22). ( k ) Systolic (SBP), diastolic (DBP) and mean (MBP) blood pressure in non-fasting WT mice and G9EKO ( n =9, 17). * P <0.05, ** P <0.01 and *** P <0.001 versus WT (two-tailed t -testing). Error bars represent s.e.m. Full size image Table 2 Indirect calorimetric data from 8- and 16-week-old wild type and G9EKO mice. Full size table We next assessed whether blocking uric acid production could reverse any of these effects of impaired urate clearance. WT and G9EKO mice were thus exposed to 8-week allopurinol (150 mg l −1 ) ad libitum in sterilized drinking water approximately 4 weeks after weaning [4] . Plasma uric acid was significantly decreased in G9EKO mice following allopurinol treatment without significant effects on urine urate concentrations ( Fig. 3a,b ). Strikingly, in comparison with untreated G9EKO mice, allopurinol treatment also lowered blood pressure and total cholesterol ( Fig. 3c,d ) without significant effects on free fatty acids and triglycerides suggesting at least partial allopurinol reversibility of the spontaneous metabolic syndrome in G9EKO mice—either through xanthine oxidase inhibition or through direct effects on renal uric acid transporters by allopurinol or by its active metabolite, oxypurinol. Fasting free fatty acid and triglyceride were not significantly affected by allopurinol ( Fig. 3e,f ). 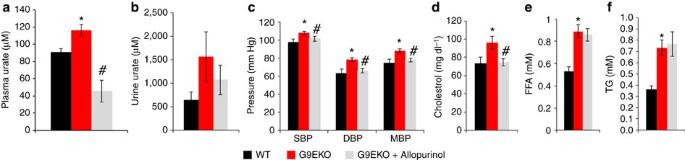Figure 3: Allopurinol mitigates G9EKO hyperuricaemia, hypertension and dyslipidaemia. (a,b) Serum (n=8, 18, 8) and urine uric acid (n=4, 7, 7) in WT and G9EKO fed sterile water or water containing allopurinol. (c) Systolic (SBP), diastolic (DBP) and mean (MBP) blood pressure in unmedicated or in allopurinol-treated G9EKO and WT mice (n=5, 9, 7). (d–f) Fasting cholesterol (n=6, 5, 8), free fatty acid (FFA) (n=5, 5, 5) and triglyceride (TG) (n=5, 5, 10) in WT and G9EKO mice. *P<0.05 versus WT.#P<0.05 versus untreated G9EKO mice (two-tailedt-testing with Bonferroni–Dunnpost hoccorrection for data sets on which multiple comparisons are made). Error bars represent s.e.m. Figure 3: Allopurinol mitigates G9EKO hyperuricaemia, hypertension and dyslipidaemia. ( a , b ) Serum ( n =8, 18, 8) and urine uric acid ( n =4, 7, 7) in WT and G9EKO fed sterile water or water containing allopurinol. ( c ) Systolic (SBP), diastolic (DBP) and mean (MBP) blood pressure in unmedicated or in allopurinol-treated G9EKO and WT mice ( n =5, 9, 7). ( d – f ) Fasting cholesterol ( n =6, 5, 8), free fatty acid (FFA) ( n =5, 5, 5) and triglyceride (TG) ( n =5, 5, 10) in WT and G9EKO mice. * P <0.05 versus WT. # P <0.05 versus untreated G9EKO mice (two-tailed t -testing with Bonferroni–Dunn post hoc correction for data sets on which multiple comparisons are made). Error bars represent s.e.m. Full size image We then looked at well-described secondary complications of hyperuricaemia in G9EKO mice, including non-alcoholic fatty liver disease and cardiovascular disease. Consistent with findings of increased steatosis/non-alcoholic fatty liver disease in patients with hyperuricaemia [16] , hepatic triglycerides and free fatty acids were elevated in G9EKO livers versus WT livers ( Fig. 4a,b ). In addition, mRNA for sterol regulatory element-binding protein, a marker of cholesterol metabolism, was significantly elevated in the livers of G9EKO mice, and there was a trend toward elevated collagen type 1 alpha and fatty acid synthase, markers of fibrosis and fat synthesis. 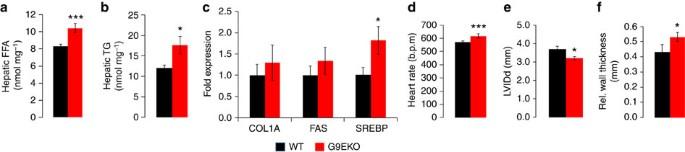Figure 4: Early-onset non-alcoholic fatty liver disease (NAFLD) and cardiac remodeling in G9EKO mice. (a,b) Hepatic free fatty acid (FFA) (n=6, 6) and triglyceride (TG) (n=6, 6) in WT and G9EKO liver homogenates. (c) Relative mRNA abundance of collagen type 1a, fatty acid synthase and sterol response element-binding protein-1 by quantitative reverse transcriptase (qRT–PCR) analysis. (d–f) Echocardiographic analysis of heart rate, diastolic left ventricular internal diameter and relative wall thickness in WT and G9EKO mice (n=5, 5). *P<0.05 versus WT. ***P<0.001 versus WT (two-tailedt-testing). Error bars represent s.e.m. Figure 4: Early-onset non-alcoholic fatty liver disease (NAFLD) and cardiac remodeling in G9EKO mice. ( a , b ) Hepatic free fatty acid (FFA) ( n =6, 6) and triglyceride (TG) ( n =6, 6) in WT and G9EKO liver homogenates. ( c ) Relative mRNA abundance of collagen type 1a, fatty acid synthase and sterol response element-binding protein-1 by quantitative reverse transcriptase (qRT–PCR) analysis. ( d – f ) Echocardiographic analysis of heart rate, diastolic left ventricular internal diameter and relative wall thickness in WT and G9EKO mice ( n =5, 5). * P <0.05 versus WT. *** P <0.001 versus WT (two-tailed t -testing). Error bars represent s.e.m. Full size image The increased incidence of cardiovascular morbidity in hyperuricaemic patients prompted us to survey the cardiac phenotype of G9EKO mice. Basal heart rate observed by echocardiography was significantly elevated in G9EKO mice ( Fig. 4d ). Echocardiogram also revealed evidence of cardiac hypertrophic remodelling, ( Fig. 4e,f )—decreased diastolic left ventricular internal diameter with increased relative wall thickness—a common finding in patients with hyperuriceamia [17] . However, although allopurinol treatment significantly lowered body weight ( Fig. 5a ) and hepatic triglyceride content ( Fig. 5c ) associated with a trend toward lower body fat mass in G9EKO mice ( Fig. 1b ), allopurinol treatment did not significantly reverse the G9EKO-associated changes in heart rate, left ventricular internal diameter or relative wall thickness ( Fig. 5d–f ). 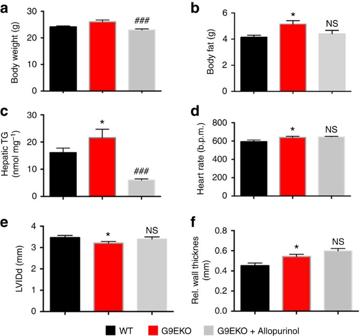Figure 5: Allopurinol reduces body weight and hepatic triglycerides in G9EKO mice. Shown is the effect of ~8-week allopurinol treatment (150 mg l−1fedad libitumin water) on (a) body weight and (b) body fat (n=21, 19, 24) and (c) hepatic triglycerides (triglyceride (TG),n=11, 9, 7). Panelsd,e,f, demonstrate the effect of allopurinol on echocardiographic parameters (n=12, 6, 12). HR, heart rate, LVIDd, internal left ventricular diameter in diastole, RWT, relative wall thickness. *P<0.05 versus WT control by two-tailedt-test after Bonferroni–Dunnpost hoccorrection for multiple comparisons.###P<0.001 versus untreated G9EKO mice. NS, not statistically significantly different versus G9EKO untreated mice (two-tailedt-test after Bonferroni–Dunnpost hoccorrection). Error bars represent s.e.m. Figure 5: Allopurinol reduces body weight and hepatic triglycerides in G9EKO mice. Shown is the effect of ~8-week allopurinol treatment (150 mg l −1 fed ad libitum in water) on ( a ) body weight and ( b ) body fat ( n =21, 19, 24) and ( c ) hepatic triglycerides (triglyceride (TG), n =11, 9, 7). Panels d , e , f , demonstrate the effect of allopurinol on echocardiographic parameters ( n =12, 6, 12). HR, heart rate, LVIDd, internal left ventricular diameter in diastole, RWT, relative wall thickness. * P <0.05 versus WT control by two-tailed t -test after Bonferroni–Dunn post hoc correction for multiple comparisons. ### P <0.001 versus untreated G9EKO mice. NS, not statistically significantly different versus G9EKO untreated mice (two-tailed t -test after Bonferroni–Dunn post hoc correction). Error bars represent s.e.m. Full size image Mice lacking enterocyte Glut9 thus develop early-onset spontaneous hyperuricaemic metabolic syndrome that is partially mitigated by allopurinol, a xanthine oxidase inhibitor. Not all deleterious findings in the G9EKO model were reversed by allopurinol, suggesting either (a) some metabolic syndrome components occur independently of hyperuricaemia, (b) some metabolic syndrome components caused by hyperuricaemia are irreversible once clinically apparent or (c) uric acid is unrelated to any findings, and the allopurinol effects are derived specifically from blocking oxidant production via xanthine oxidase inhibition per se . It should be noted, however, that the key advantage to this model of impaired urate excretion in delineating the specific effects of hyperuricaemia is that it does not rely on xanthine oxidase activity to produce hyperuricaemia as in some of the diet-induced models (for example, fructose- or purine-rich diets). Nevertheless, while further insight into the effects of hyperuricaemia on its host are required, the G9EKO model suggests that attenuated enterocyte urate clearance could be a critical, initiating step in metabolic syndrome pathogenesis. Interdicting circulating urate accumulation by focusing on gut urate reuptake and clearance could represent a novel treatment paradigm to block or modulate hyperuricaemia and its complications, including metabolic syndrome. We expect this model can now be used to probe mechanistically into the role of urate in the complications and sequelae of metabolic syndrome. Generation of G9EKO Mice Enterocyte-specific Glut9-deficient mice were generated by homologous recombination of the 18.9 kb targeting vector harbouring loxP sites flanking exons 5 and 6 and a neomycin resistance cassette 3′ of exon 6. Modified embryonic stem cells from 129Sv mice carrying this targeting allele were introduced into C57BL/6 blastocysts. Chimeric offspring were twice backcrossed into the C57BL/6 line to generate N2 mice heterozygous for the targeting allele (genotype Slc2a9 fl/+ ). N2 mice were intercrossed to generate homozygous ( Slc2a9 fl/fl ) mice. Genotyping primers were as follows (listed 5′–3′): forward primer—5′-TGGTGCTACTCTGTGGTGCTA-3′; reverse primer—5′-CACAGCGGTGAAAGTAACGA-3′. Mice harbouring homozygous floxed Slc2a9 alleles were crossed with mice expressing Cre recombinase under the mouse villin 1 promoter on a C57/BL6 background (Jackson Laboratories, stock number 004586) to generate G9EKO mice. Mice expressing villin promoter-driven Cre with WT Slc2a9 alleles were used as control mice throughout these studies. For allopurinol treatment experiments, 8-week-old mice were maintained on 150 mg l −1 allopurinol [4] for 8 weeks before metabolic characterization. All animal procedures were approved by the Washington University School of Medicine Animal Studies Committee. Calorimetry body composition and blood pressure determination Indirect calorimetry, echoMRI and blood pressure analyses on unanaesthetized mice were performed via the Mouse Diabetic Models Phenotyping Core Facility at Washington University using an Oxymax Indirect Calorimeter (Columbus Instruments, Columbus, OH, USA), an EchoMRI 3–1 (Echo Medical Systems, Houston, TX, USA [18] , [19] and a Columbus Instruments NIBP (Columbus) tail-cuff and plethysmograph. Food consumed in mice was measured in 24-h increments during each calorimetry run. Radiolabelled uric acid uptake measurements Apical villous enterocytes first were enriched by calcium chelation and mechanical disruption [20] . Briefly, sections of distal jejunum (5–6 cm) were removed, flushed with ice-cold phosphate-buffered saline and opened longitudinally before immersion in ice-cold phosphate-buffered saline. The bowel was transferred into 5 ml ice-cold balanced salt solution (BSS) buffer (1.5 mM KCl, 96 mM NaCl, 27 mM sodium citrate, 8 mm KH 2 PO 4 , 5.6 mM Na 2 HPO 4 , 15 mM EDTA, and 1 mM dithiothreitol) and vortexed at 4 °C at maximum speed for 20 min. Following this step, almost all epithelial cells were recovered in the BSS solution. The BSS solution (containing crypts and villi) was filtered through a 70-μm cell strainer (BD Biosciences, San Jose, CA, USA). The larger size villi were captured in the cell strainer whereas crypts were discarded in the effluent. Crypt fractions were then spun down at 1,000 g for 10 min at 4 °C and washed once with Tris buffer (150 mM NaCl, 1 mM EDTA, 1 mM EGTA, 50 mM Tris-HCl, pH 8.0) then with ice-cold DMEM before assay. To assay uptake, cells were resuspended in pre-warmed, 37 °C DMEM containing 1 μCi ml −1 [ 14 C]-uric acid (American Radiolabeled Chemicals, St Louis, MO, USA) for 3 min before quenching and three wash steps in ice-cold Hank’s balanced salt solution. Samples were subjected to liquid scintillation counting and counts were normalized to sample protein, as determined by bicinchoninic acid assay kit (Pierce, Rockford, IL, USA). Western Blotting and immunostaining Western blotting was performed using 50–100 μg protein subjected to 10% SDS–PAGE, followed by transfer to nitrocellulose membrane and overnight primary antibody incubation [21] , [22] (1:1,000 dilutions at 4 °C) with the following antisera: total Glut9, glyceraldehyde 3-phosphate dehydrogenase (clone 14C10, Cell Signaling Technologies, Beverly, MA, USA), Glut9A [12] Actin (clone C4, EMD Millipore, Billerica, MA, USA). Fixed (4% paraformaldehyde), paraffin-embedded intestinal sections were sectioned, permeablized in 0.1% Triton X-100 in phosphate-buffered saline and blocked with 2% bovine serum albumin (Sigma-Aldrich, St Louis, MO, USA) before immunostaining using pre-immune serum or GLUT9-specific antibody (Generated in the laboratory of Dr Annette Schürmann) at a 1:200 dilution. LC and tandem mass spectrometry Uric acid analysis in stool was performed by the Washington University Metabolomics Facility. Uric acid was extracted from ~20 mg dried, pulverized, sieved mouse stool using water containing 1-methyluric acid (Sigma) for LC/MS/MS using a modified US analysis method [22] . 1-methyluric acid was chosen as the internal standard and a Thermo betasil LC column was used for negative ion electrospray LC/MS/MS analysis. Hepatic lipid extraction Hepatic lipids were extracted by homogenizing 100 mg of liver tissue in 2 ml (2:1) chloroform:methanol [23] . Remaining tissue was pelleted by centrifugation and 10–20 μl supernatant aliquots were dried for 2 h before resuspension in assay reagent. Values were normalized to tissue input mass. Biochemical analyses Serum and urine uric acid, serum and hepatic cholesterol, triglyceride, free fatty acid and serum insulin were measured using the following kits precisely per the manufacturer’s instructions [18] , [19] , [23] : Amplex Red Uric Acid Assay Kit (Invitrogen, Carlsbad, CA, USA), Infinity Cholesterol Assay Kit, (Thermo Scientific, Waltham, MA, USA), Infinity triglyceride assay kit (Thermo Scientific, Waltham, MA, USA), NEFA free fatty acid determination kit (Wako Diagnostics, Richmond, VA, USA) and rat/mouse insulin ELISA assay kit (Millipore, Billerica, MA, USA). Echocardiography Echocardiography was performed by the Washington University Mouse Cardiovascular Phenotyping Core Facility [21] . Non-invasive transthoracic cardiac ultrasound exams were performed under light general anaesthesia using a VisualSonics Vevo 2100 cardiac echocardiography machine with a 15-MHz linear transducer. Statistical analysis All values are expressed as the mean±s.e.m. Two-tailed t -tests were applied with Bonnferroni–Dunn post hoc correction for multiple comparisons. P <0.05 was considered to be statistically significant between groups. How to cite this article: DeBosch, B. J. et al. Early-onset metabolic syndrome in mice lacking the intestinal uric acid transporter SLC2A9 . Nat. Commun. 5:4642 doi: 10.1038/ncomms5642 (2014).